Stretchable batteries with self-similar serpentine interconnects and integrated wireless recharging systems An important trend in electronics involves the development of materials, mechanical designs and manufacturing strategies that enable the use of unconventional substrates, such as polymer films, metal foils, paper sheets or rubber slabs. The last possibility is particularly challenging because the systems must accommodate not only bending but also stretching. Although several approaches are available for the electronics, a persistent difficulty is in power supplies that have similar mechanical properties, to allow their co-integration with the electronics. Here we introduce a set of materials and design concepts for a rechargeable lithium ion battery technology that exploits thin, low modulus silicone elastomers as substrates, with a segmented design in the active materials, and unusual ‘self-similar’ interconnect structures between them. The result enables reversible levels of stretchability up to 300%, while maintaining capacity densities of ~1.1 mAh cm −2 . Stretchable wireless power transmission systems provide the means to charge these types of batteries, without direct physical contact. Development of classes of electronic and optoelectronic technologies that offer elastic responses to large strain (»1%) deformations has accelerated in recent years [1] , [2] , [3] , [4] , [5] , [6] . Combinations of materials, device layouts, mechanics designs and manufacturing approaches are now beginning to emerge for realistic applications in areas ranging from wearable photovoltaics [7] to ‘epidermal’ health/wellness monitors [8] , to sensitive robotic skins [9] , [10] , [11] to soft surgical tools [12] and electronic ‘eyeball’ imaging devices [13] . In all cases, stretchability represents a key, enabling characteristic. For many of these and other uses, a critical need lies in energy-storage devices with similar physical properties, to allow for direct and natural integration with the electronics [14] . Many important storage devices have been developed with flexible characteristics, including supercapacitors [15] , [16] , [17] and batteries [17] , [18] , where sufficiently thin geometrical forms lead to flexibility, by virtue of bending-induced strains (typically to values of ~1% or less) that decrease linearly with thickness, for a given bend radius. Stretchability, on the other hand, represents a more challenging type of mechanics, in which the systems must accommodate large strain deformation (»1%), typically of arbitrary form, including not only bending, but also twisting, stretching, compressing and others, and thickness is typically not a critical factor. Stretchable supercapacitors using buckled thin films of carbon nanotubes (CNTs) [19] or CNT-soaked fibrous textiles [20] , and stretchable non-rechargeable zinc carbon batteries based on conductive fabrics [21] , [22] represent two examples. Although these technologies each have attractive features, none offers multiple capabilities in recharging with high-storage capacity, stretching to large levels of deformation (>100%), or establishing wireless electrical interfaces to external power supplies. The materials and integration schemes reported here achieve these characteristics in a type of lithium ion battery that exploits segmented layouts and deformable electrical interconnects in specialised, ‘self-similar’ geometries. The resulting devices offer biaxial stretchability up to strains of 300%, with capacity densities of ~1.1 mAh cm −2 , and little loss in capacity for up to 20 cycles of recharging. The designs also allow integration of stretchable, inductive coils to enable charging through external supplies without the need for physical connexions. This set of attributes satisfies requirements for many applications that are being contemplated for stretchable electronics. Battery design The devices exploit pouch cells in which arrays of small-scale storage components are connected by conducting frameworks with extraordinary stretchable characteristics. A schematic illustration of the system, an exploded view of the multilayer construction of a unit cell, and a representation of the ‘self-similar’ interconnect geometries appear in Fig. 1a–c , and Supplementary Fig. S1 . The current collectors consist of photolithographically patterned circular disks of aluminium (600 nm) and copper (600 nm). Layers of polyimide (PI; 1.2 μm) encapsulate interconnecting traces between these disks in a way that places the metals close to the neutral mechanical plane ( Fig. 1d , left panel). Thin (0.25 mm), low modulus (60 kPa) sheets of silicone elastomer form top and bottom substrates that support these structures ( Fig. 1d , middle panel) and other components of the batteries. The overall construct consists of a square array of 100 electrode disks, electrically connected in parallel. Moulded pads of slurries based on LiCoO 2 and Li 4 Ti 5 O 12 serve as active materials at the cathode and anode [23] , [24] , respectively ( Fig. 1d , right panel, and Supplementary Fig. S2 ). The two sheets laminate together in a way that involves spatial offsets between the active materials to avoid electrical shorts between them and to eliminate the need for a separator. A spacer, made of the same silicone elastomer and applied around the periphery of the system, prevents direct contact of the top and bottom sheets. A gel electrolyte injected into the gap provides media for ionic transport. Thin encapsulating layers of an acryloxy perfluoropolyether elastomer bonded to the outer surfaces help to prevent moisture from diffusing into the battery and solvents in the gel from leaking out [25] . Long-term operation requires more sophisticated packages consisting of for example, buckled bilayer sheets of aluminium/PI that bond to the outer surfaces of the battery ( Supplementary Fig. S3 ). The materials and fabrication details appear in the Methods section. 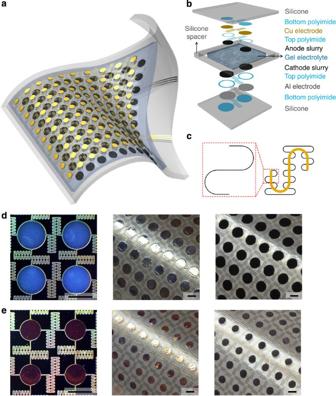Figure 1: Aspects in battery layout and design. (a) Schematic illustration of a completed device, in a state of stretching and bending. (b) Exploded view layout of the various layers in the battery structure. (c) Illustration of ‘self-similar’ serpentine geometries used for the interconnects (black: 1st level serpentine; yellow: 2nd level serpentine). (d) Optical images of the Al electrode pads and self-similar interconnects on a Si wafer (left panel; top down view; ~4 unit cells), after transfer printing on a sheet of silicone (middle panel; top down view, in a bent geometry), and with moulded slurries of LiCoO2(right panel; top down view, in a bent geometry). (e) Optical images of the Cu electrode pads and self-similar interconnects on a Si wafer (left panel; top down view; ~4 unit cells), after transfer printing on a sheet of silicone (middle panel; top down view, in a bent geometry), and with moulded slurries of Li4Ti5O12(right panel; top down view, in a bent geometry). Scale bars indandeare 2 mm. Figure 1: Aspects in battery layout and design. ( a ) Schematic illustration of a completed device, in a state of stretching and bending. ( b ) Exploded view layout of the various layers in the battery structure. ( c ) Illustration of ‘self-similar’ serpentine geometries used for the interconnects (black: 1st level serpentine; yellow: 2nd level serpentine). ( d ) Optical images of the Al electrode pads and self-similar interconnects on a Si wafer (left panel; top down view; ~4 unit cells), after transfer printing on a sheet of silicone (middle panel; top down view, in a bent geometry), and with moulded slurries of LiCoO 2 (right panel; top down view, in a bent geometry). ( e ) Optical images of the Cu electrode pads and self-similar interconnects on a Si wafer (left panel; top down view; ~4 unit cells), after transfer printing on a sheet of silicone (middle panel; top down view, in a bent geometry), and with moulded slurries of Li 4 Ti 5 O 12 (right panel; top down view, in a bent geometry). Scale bars in d and e are 2 mm. Full size image The devices must accommodate two competing design goals: (1) high areal capacity, which requires large coverage of the active regions, and (2) high mechanical stretchability, which requires large distances between these regions. Strategic features of relief on the elastomer substrates provide a partial solution to this challenge, as demonstrated recently in photovoltaic modules [26] , [27] . A disadvantage is that levels of stretchability beyond ~30% can be difficult to achieve without sacrificing coverage. Here, we take a different, but complementary, approach in which the focus is on deformable interconnects with advanced designs. In particular, we introduce layouts that use ‘self-similar’ structures of wires in serpentine configurations to offer, simultaneously, high system-level stretchability, and low interconnect resistances. A conventional serpentine consists of circular arcs connected by straight lines. ‘Self-similar’ designs follow from iteratively applying this basic geometry, beginning with a unit cell as illustrated schematically in the red box of Fig. 1c . Here, reducing the scale of the cell, and then connecting multiple copies of it in a fashion that reproduces the layout of the original cell geometry, corresponds to one iteration. The yellow line in Fig. 1c represents a 2nd order serpentine geometry, created in this manner. Although higher orders can be designed and implemented easily, the 2nd order construct satisfies requirements for the applications considered here, as described in detailed experimental and theoretical study below. Mechanical characteristics of the ‘self-similar’ interconnects Three-dimensional finite element analysis (see Supplementary Methods ) and experimental measurements illustrate the essential mechanics. Test samples fabricated for this purpose consist of free-standing, multilayer traces, with materials and multilayer stack designs (PI (1.2 μm)/Cu (0.6 μm)/PI (1.2 μm)) that match those used in the batteries, between circular pads that bond to posts moulded onto underlying elastomer substrates. The self-similar geometry leads to hierarchical buckling physics that ensures ultra-low strains in the materials, even under extreme stretching [3] , [28] . For the entire range of tensile strains examined, from 0 to 300%, the configurations predicted by FEA agree remarkably well with optical images collected during the experiments, as shown in Fig. 2 and Supplementary Movies 1 and 2 . Both symmetric and anti-symmetric buckling modes exist (see Supplementary Fig. S4 for detailed illustrations of the two modes). The trace consists of three columns of serpentine wires connected by two horizontal straight lines. We refer to the construct that corresponds to the ‘short’ wavelength serpentine within each column as the 1st level; the 2nd level corresponds to the large-scale serpentine shape, with ‘long’ wavelength. For the symmetric buckling mode ( Supplementary Fig. S4a ), the left and right columns undergo mainly an overall bending deformation along the vertical direction, resulting in the collective upward motion of the entire middle column of serpentine wires. In this sense, the out-of-plane displacement is symmetric with respect to the centre line ( x =0) in the ‘Front view’ of Supplementary Fig. S4a . For the anti-symmetric buckling mode ( Supplementary Fig. S4b ), the serpentines in the left and right columns mainly undergo an overall twisting deformation along the vertical direction. Here, the two ends of middle serpentine move in opposite directions (that is, one moves up, and the other moves down). In this case, the out-of-plane displacement is anti-symmetric with respect to the centre line ( x =0) in the ‘Front view’ of Supplementary Fig. S4b . The critical buckling strains obtained by FEA for the symmetric (0.078%) and anti-symmetric (0.087%) modes are much lower than those (>0.172%) for all other buckling modes. This result is consistent with experimental observation of only these two modes. In both cases, the physics associated with stretching involves a mechanism of ‘ordered unravelling’, which begins at the 2nd level, at a well-defined, critical buckling strain, ~0.08% for the example investigated here. Next, the 2nd level gradually ‘unravels’ via bending and twisting as the applied strain increases from 0.08% to ~150%, during which there is essentially no further deformation in the 1st level. The motions in the 1st level start when the 2nd level is almost fully extended, corresponding to an applied strain of ~150% in this case. As the ‘unravelling’ of the 1st level serpentine approaches its end, the strain in the materials begin to increase rapidly, thereby defining the practical limit in stretchability. 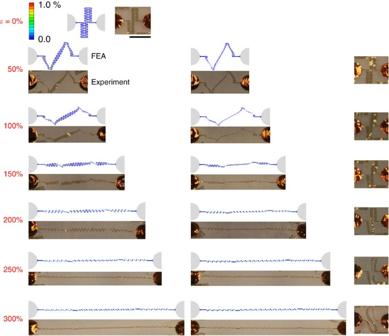Figure 2: Experimental and computational studies of buckling physics in interconnects with self-similar serpentine layouts. Optical images and corresponding finite element analysis (FEA) of symmetric (left column) and anti-symmetric (middle column) deformation modes, for various levels of applied tensile strain (ε). The colour in the FEA results represents the maximum principal strains of the metal layer. The scale bar is 2 mm. The right column shows the interconnect structures after releasing the applied strain. Figure 2: Experimental and computational studies of buckling physics in interconnects with self-similar serpentine layouts. Optical images and corresponding finite element analysis (FEA) of symmetric (left column) and anti-symmetric (middle column) deformation modes, for various levels of applied tensile strain ( ε ). The colour in the FEA results represents the maximum principal strains of the metal layer. The scale bar is 2 mm. The right column shows the interconnect structures after releasing the applied strain. Full size image For applied strains below this limit, the deformation mechanisms of ordered unravelling processes ensure low levels of strain in the materials ( Supplementary Fig. S5 ). For a representative failure strain of 1% for copper, FEA predicts a stretchability of 321%, which is in good agreement with the experimental observations (300%< ε stretchability <350%) (simulations suggest that the copper reaches its failure point before the PI). For reversible behaviour (that is, the interconnects return to their initial configuration after release), the maximum material strain must be less than the yield strain. For a representative yield strain of 0.3% for copper, FEA suggests reversibility for applied strains up to ~168%. This value is lower than experimental observations, where reversibility occurs even for strains of between 200% and 250% ( Fig. 2 ). The likely explanation for this discrepancy is that yield occurs first in only small portions of the interconnect (for example, one element in the FEA). In this case, the effects on reversibility might not be easily observed in experiments. These levels of stretchability (>300%) and reversibility (>200%) significantly exceed those of previous reports in stretchable batteries and/or battery electrodes; they are also greater than those of any other reports of stretchable interconnects that use lithographically defined patterns of conventional metals. The importance of the self-similar designs can be assessed through comparisons of stretchability to otherwise similar, but conventional serpentine structures: the former exhibits a stretching range of 321%, while the latter is 134%, determined by FEA ( Supplementary Fig. S6 ). Furthermore, even for the same total length ( l total ), span ( L ), amplitude ( h ), and cross-section (width w and thickness t ), the self-similar design again outperforms the conventional serpentine, both in stretchability (809% versus 682%) and reversibility (528% versus 284%) ( Supplementary Fig. S7 ). We note that in all cases of uniaxial stretching, the Poisson effect leads to compression in the orthogonal direction. The buckling profiles in these regions have behaviours that are consistent with FEA ( Supplementary Fig. S8 ). Electrochemical and mechanical behaviour of the battery After choosing a set of dimensions that offers excellent system-level stretchability, with good areal capacity density, and modest interconnect resistance, we observed the best electrical performance for layouts in which the diameters of the disks for the cathode and anode are 2.20 mm and 1.58 mm, respectively, and the offset distances are 0.51 mm. This configuration corresponds to an areal coverage of 33% for the cathode, 17% for the anode, and 50% for the entire battery (in the undeformed configuration) ( Supplementary Fig. S9 ). The interconnects have thicknesses of 600 nm and widths of 50 μm. For these parameters, the resistance between adjacent disks is 24 Ω, and that between the connexion lead and the most distant disk is 45 Ω. The leads for external connexion are thin and narrow to avoid strain at the interface, and facilitate connexion to flexible (but not stretchable) cables that connect to external characterisation equipment. The gel electrolyte combines the flow properties of viscous liquids with the cohesive properties of a solid, thereby allowing it to accommodate large strains while maintaining ionic conduction pathways. Electrochemical properties of the battery electrodes without and with 300% uniaxial strain appear in Fig. 3a . The results show two well-defined plateaus at around 2.35 V corresponding to potentials of Co 3+ / 4+ and Ti 4+ / 3+ redox couples [29] . The mass of the LiCoO 2 (specific capacity 145 mAh g −1 ) at each unit is ~95 mg, and thus areal capacity density of 1.1 mAh cm −2 at a charge/discharge rate of C/2. The mass of Li 4 Ti 5 O 12 (specific capacity 160 mAh g −1 ) is ~90 mg, which corresponds to 5–10% more anode capacity than cathode [30] . Slurry disks with thicknesses larger than those described here yield improved areal capacity density, but with reduced rate capability due to the concentration polarisation in the disks [31] , [32] . The output resistance of the battery is ~70 Ω ( Supplementary Fig. S10 ), and the leakage current is 1–10 μA, which arises from two main sources: the internal ohmic self-discharge between the slurry disks at the anode and cathode and Faradaic effects, including shuttle reactions associated with impurities in the slurry materials, residual oxygen and/or moisture. Experimental measurements described in the Supplementary Methods and Supplementary Fig. 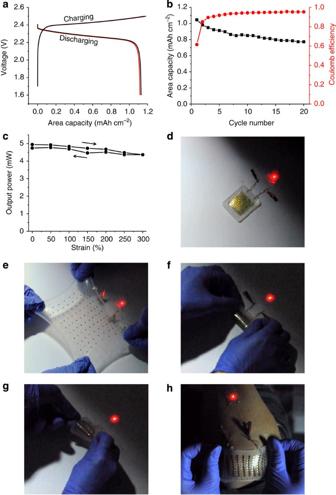Figure 3: Electrochemical and mechanical properties of the battery. (a) Galvanostatic charging and discharging of the battery electrodes without (black) and with 300% uniaxial strain (red). (b) Capacity retention (black) and coulombic efficiency (red) over 20 cycles with a cutoff voltage of 2.5–1.6 V. (c) Output power as a function of applied biaxial strain. (d) Operation of a battery connected to a red light-emitting diodes (LED) while (e) biaxially stretched to 300%, (f) folded, (g) twisted and (h) mounted on the human elbow. S11 show that use of separators and enhanced packaging schemes can reduce the capacity loss from 161 μA h to 23 μA h in 44 h. Figure 3b shows the coulombic efficiency (red) and cycling performance (black) of the encapsulated battery. The coulombic efficiency rises from ~60% for the first cycle to over 90% after three cycles. The initial loss can be attributed to the formation of a solid-electrolyte-interphase, and lithium is consumed in side reactions with impurities in the electrolyte. The gradually degrading capacity retention results not from the cycle fade ( Supplementary Fig. S12 ) but more likely from the calendar fade due to some combination of reaction with residual water in the packaging materials, moisture penetration and electrical discontinuity of slurry particles that detach from the disks, which are not hot pressed and can be sometimes observed in the electrolyte gel. Further increasing the baking temperature and optimising the composition of the slurries, such as increasing the binder ratio, could reduce the latter behaviours. Improved conditions for device assembly could reduce effects of the former. Varying the depth of discharge from 100% to 75% did not have a significant effect on the degradation characteristics ( Supplementary Fig. S13 ). Figure 3c shows the output power of the battery, when connected to a resistor 2.02 kΩ), during biaxial stretching and releasing. The slight decrease in output power with strain likely results from increased internal resistances that arise from the significantly increased separations between slurry disks with strains at these large levels. The battery provides sufficient power to operate commercial light-emitting diodes, with turn on voltages of 1.7 V ( Supplementary Fig. S14 ), as shown in Fig. 3d . The battery could be stretched by up to 300% ( Fig. 3e , Supplementary Movie 3 ), folded ( Fig. 3f ) and twisted ( Fig. 3g ) without noticeable dimming of the light-emitting diode. Furthermore, FEA demonstrates that the effective modulus (66.8 kPa) of the full composite structure of the battery is only slightly higher than the modulus (60.0 kPa) of the silicone substrate materials. As a result, the battery is not only stretchable but also exceptionally soft and compliant. The battery modulus is, in fact, lower than that of the human epidermis (140–600 kPa) [8] , thereby offering the potential for integration onto the skin and biological tissues, without significant mechanical loading. Figure 3h shows that the battery is compliant when mounted on human skin. Figure 3: Electrochemical and mechanical properties of the battery. ( a ) Galvanostatic charging and discharging of the battery electrodes without (black) and with 300% uniaxial strain (red). ( b ) Capacity retention (black) and coulombic efficiency (red) over 20 cycles with a cutoff voltage of 2.5–1.6 V. ( c ) Output power as a function of applied biaxial strain. ( d ) Operation of a battery connected to a red light-emitting diodes (LED) while ( e ) biaxially stretched to 300%, ( f ) folded, ( g ) twisted and ( h ) mounted on the human elbow. Full size image Stretchable wireless charging system for the battery In many practical cases such as implanted devices the ability to charge the battery without establishing physical connexions to external supplies can be valuable. Even in systems where the charging terminals are accessible, such as in skin-mounted systems there is value in wireless charging, simply because the process of establishing physical contacts can be mechanically destructive to thin, stretchable components (or to the underlying soft tissue). Approaches that involve physical contact also have the danger of electrical shock to surrounding materials (for example, the skin itself). The versatility of the materials and designs enable integration of wireless power transmission systems, monolithically with the battery itself. The design and an actual device appear in Fig. 4a and b , respectively. A secondary coil couples the electromagnetic flux from a primary coil, and a Schottky diode provides rectification. The Schottky diode (packaged in epoxy, with a modulus of ~4.0 GPa) has a modulus of more than 4 orders of magnitude larger than that of the silicone substrate, but its size (length 0.62 mm, width 0.32 mm and height 0.31 mm) is only a few per cent (~2%) of the overall size (~30 mm × ~20 mm) of the wireless system. As a result, the influence on the overall stretchability is still negligible, as demonstrated by finite element simulations shown in Supplementary Figs S15 and S16 . The parallel capacitor smooths oscillations in the output voltages; its small size and thickness enable natural integration into the overall system. Larger capacitors can smooth the oscillations to an even greater extent ( Supplementary Fig. S17 ). The coil and rectifier add a series resistance of 2.3 kΩ ( Supplementary Fig. S18 ), which functions as a parallel resistance with the secondary coil, shunting away current from the battery. The resistance of the serpentine secondary coil is 1.92 kΩ m −1 ; a coil with similar overall geometry but without the serpentine shape is calculated to be 1.22 kΩ m −1 . The efficiency of the charging system can be improved by increasing the width and thickness of the wires, but at the expense of reduced stretchability and increased modulus. Specific application requirements will define the right tradeoffs. In this case, the output power from the primary coil was 187 mW. With a working distance of 1 mm between the primary and secondary coil, the power received on the secondary coil is 9.2 mW, corresponding to an efficiency of 4.9%. Increasing the secondary coil thickness to 7 μm improves the efficiency from 4.9 to 17.2%. At this thickness, the coil retains stretchability to strains of 25% ( Supplementary Fig. S19 ). The capacitor has a capacitance of 1.7 nF, in a structure that uses a 1.2-μm thick layer of PI as the dielectric, with a layer of thiol molecules on the bottom Au electrodes to enhance adhesion. 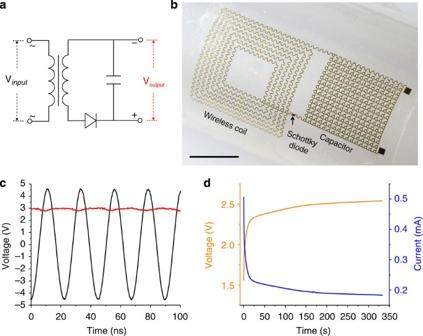Figure 4: Stretchable system for wireless charging. (a) Circuit diagram. (b) Image of the integrated system with different components labelled. (c) Characterisation of the wireless coil with an alternating voltage input at a frequency of 44.5 MHz (black) and the resulting direct voltage output (red), as indicated ina. (d) Charging voltage (orange) and current (blue) curves as a stretchable battery is charged with 3 V output from the wireless circuit. The scale bar inbis 1 cm. Figure 4c shows the input and output of this wireless power transmission device. An input voltage at a frequency of 44.5 MHz matches the self-resonant frequency of the secondary coil, which depends on the coil area, number of turns, distance between each turn and wire resistance. For a peak-to-peak input voltage of 9.1 V ( Fig. 4c , black curve), the DC output voltage is 3.0 V ( Fig. 4c , red curve). The charging curves of a small-scale battery using the wireless coil appear in Fig. 4d . The battery voltage ( Fig. 4d , orange curve) rises to 2.5 V in about 6 min. The charging current in the circuit ( Fig. 4d , blue curve) decreases from 0.5 mA to below 0.2 mA. We used a partial differential equation to model the charging circuit, and a numerical program to calculate the charging current curve. Simulation of this process agrees well with the experimental data (see Supplementary Methods and Supplementary Fig. S20 ). Figure 4: Stretchable system for wireless charging. ( a ) Circuit diagram. ( b ) Image of the integrated system with different components labelled. ( c ) Characterisation of the wireless coil with an alternating voltage input at a frequency of 44.5 MHz (black) and the resulting direct voltage output (red), as indicated in a . ( d ) Charging voltage (orange) and current (blue) curves as a stretchable battery is charged with 3 V output from the wireless circuit. The scale bar in b is 1 cm. Full size image The materials and schemes reported here provide routes to energy-storage devices and wireless charging systems with forms and properties that are attractive for powering stretchable electronic and optoelectronic devices. The slurry materials themselves are deployed in ways (a soft lithographic type casting process) that allow natural integration with unusual materials (low modulus silicone rubber sheets, possibly embossed with surface relief). The stretchable interconnects exploit a ‘self-similar’ design that offers unique, ‘spring within a spring’ mechanics. The consequence is a level of stretchability that is more than × 4 larger than previous reports, even while, at the same time, enabling coverages of active materials as high as 50%. The combination of these two aspects, together with comprehensive and experimentally validated models of the underlying mechanics, leads to a technology, that is, a stretchable, rechargeable battery, which offers much different characteristics than anything that has been previously possible. As an additional advance, we introduce integrated stretchable, wireless charging systems that offer physical properties similar to those of the batteries. Improvements will follow from further development of slurry chemistries, separator materials, and stretchable, air-impermeable packaging materials. Wireless power transfer efficiency can be increased by reducing the input resistance, maximising the mutual inductance and increasing the self-resonant frequency of the coils. Incorporating regulation circuits to avoid over-charging and over-discharging to the battery also represents an important potential direction for future work. Fabrication of electrodes and mechanical testing of self-similar interconnects Sequential spin-casting defined a bilayer of poly(methyl methacrylate) (PMMA 495 A2, 3,000 r.p.m. for 30 s, baked on a hotplate at 180 °C for 2 min) and then a layer of PI (from poly(pyromellitic dianhydride- co -4,4′-oxydianiline) amic acid solution; 4,000 r.p.m. for 30 s, baked on a hotplate at 150 °C for 4 min and then in a vacuum oven at 10 mT and 250 °C for 1 h) on a silicon wafer. The cathode and anodes consisted of 600 nm thick layers of Al or Cu, respectively, deposited by electron beam evaporation onto the PI. Photolithography (AZ5214E) and etching (Type A aluminium etchant on hotplate at 50 °C for 2 min; Type CE-100 copper etchant at room temperature for 10 s; Transene Company) defined patterns in these metals. After removing the residual photoresist, spin coating formed an additional layer of PI over the entire structure. Next, photolithography (AZ 4620, 2,000 r.p.m. for 30 s, baked at 110 °C for 4 min) and oxygen plasma etching (300 mT, 20 sccm O 2 , 200 W for 10 min) patterned the layers of PI in a geometry matched to the metal traces. Immersion in hot acetone partially removed the underlying PMMA layer, thereby allowing the entire structure to be retrieved from the silicon wafer onto the surface of a piece of water-soluble tape (3 M). Electron beam evaporation of Ti (5 nm)/SiO 2 (50 nm) through a shadow mask formed backside coatings aligned to the metal disks [33] . Thin (250 μm) silicone substrates (Ecoflex, Smooth-On) were prepared by mixing the two components in a 1:1 weight ratio, spin-casting (300 r.p.m. for 30 s) the resulting material into a Petri dish and then partially curing it (30 min at room temperature). Next, spin-casting (3,000 r.p.m. for 30 s) an allyl amide functional perfluorinated ether (DuPont), and then curing it under ultraviolet (UV) light for 30 min formed a top encapsulation layer. The other side of the Ecoflex substrate was surface activated under UV light for 5 min. Laminating the electrode structures onto this surface led to strong bonding, upon contact [34] . The water-soluble tape was removed by immersing the substrate in tap water for overnight. As a final step, the electrodes were dipped in 1 mM HCl to remove oxides from the surfaces of the metals. Mechanical testing of the self-similar interconnects was performed with a customised uniaxial stretcher. To ensure that the interconnects were decoupled from the substrate, each disk was mounted on top of a post (250 mm in height) moulded into the silicone substrate. Images and video of the deformed interconnects were collected with a digital single-lens reflex camera. Patterned moulding of slurries and their integration with current collecting electrodes Photolithography (AZ 4620, 7–8 μm thick) and inductively coupled plasma reactive ion etching (ICP RIE) defined arrays of cylindrical wells on the surface of a silicon wafer. The conditions were chosen to yield sloped sidewalls, which are important for effective transfer of the slurries, as described subsequently. Washing with acetone removed the photoresist. A layer of polytetrafluoethylene (~200 nm) conformally deposited using the ICP RIE tool served as a coating to prevent adhesion. The slurry materials consisted of lithium cobalt oxide or lithium titanium oxide, acetylene black and polyvinylidene fluoride, mixed in a weight ratio of 8:1:1 in a solvent of N -methyl-2-pyrrolidone for the cathode and anode, respectively. The mixture was stirred for overnight, and then mechanically scraped across the etched surface of the silicon wafer. The cylindrical wells, filled with slurry in this manner, were baked on a hotplate at 90 °C for overnight, and then retrieved onto the surface of a piece of water-soluble tape. The baking conditions were selected carefully to enable retrieval of the slurry with high yield. Registering the tape to the metal electrodes ensured that the moulded slurry aligned to the metal disks. Immersion in tap water for overnight dissolved the tape. Baking the substrates at 170 °C for overnight in a vacuum oven removed the moisture and improved the strength of bonding between the slurry and the metal. Assembly and electrochemical testing of the battery Anisotropic conductive films, hot pressed onto the metal electrodes, served as points for external electrical connexion. Application of Sylgard Prime Coat (Dow Corning, Inc.) to the periphery of the substrates prepared them for bonding. A thin silicone spacer layer (500 μm thick) at the periphery prevented direct contact as the two sheets were laminated together. A lateral spatial offset prevented electrical shorting between the active regions. The edges were sealed with an additional application of Ecoflex followed by baking on a hotplate (90 °C for 2 h). The gel electrolyte consisted of a mixture of 100 g lithium perchlorate, 500 ml ethylene carbonate, 500 ml dimethylcarbonate and 10 g polyethylene oxide (4 × 10 6 g mol −1 ), prepared in an argon-filled glovebox as a homogenous gel. This material was injected into the battery using a syringe through an edge. A BioLogic VMP3 electrochemical station with a cutoff voltage of 2.5–1.6 V at room temperature was used to charge and discharge the as-fabricated and stretched battery electrodes, and to evaluate cycling behaviour of the full, integrated battery. Areal capacity density was calculated based on the active region. The output power was monitored with the battery connected to a 2020 Ω resistor, using an ammeter. Values of current were recorded as a function of strain applied to the battery. Fabrication and testing of the wireless coil A silicon wafer, coated with layers of PMMA and PI using steps described previously, served as a substrate for deposition of Cr (5 nm)/Au (500 nm) by electron beam evaporation. Photolithography (AZ 5214E) and etching (Transene Company) defined patterns in the geometry of the bottom electrode of the capacitor and associated contact lines. Removing the photoresist with acetone, and then immersing the substrate in a 1 mM poly(ethylene glycol) methyl ether thiol solution in isopropanol for 15 min served to enhance the adhesion and coverage of a second layer of PI spin-cast (4,000 r.p.m. 30 s) and cured (on hotplate at 150 °C for 4 min and then in vacuum oven at 250 °C for 1 h) on the electrodes. This layer of PI served as the dielectric for the capacitor. Photolithography (AZ 4620, 2,000 r.p.m. for 30 s, baked at 110 °C for 4 min) defined a mask for etching vias through the PI layer, as points of connexion between the coil and the bottom electrode of the capacitor. After immersion in acetone to remove the photoresist, sputter deposition formed a conformal layer of Cu (600 nm) over the entire surface, including the sidewalls of the vias. Photolithography (AZ 5214E) and etching defined the coil and the other top electrode of the capacitor. After removing the resist, a third spin-cast layer of PI formed a coating on the Cu electrodes. An oxygen plasma etching through the three PI layers in a patterned geometry defined the final device layout. Undercut by immersion in hot acetone partially removed the underlying PMMA, to enable the release of the entire structure onto water-soluble tape. Deposition of Ti (5 nm)/SiO 2 (50 nm) and lamination onto the UV-activated surface of an Ecoflex substrate led to strong bonding. After the water-soluble tape was removed, a Schottky diode chip (Digikey BAT 62-02LS E6327) was bonded between the coil and the capacitor using silver epoxy. The forward input resistance is ~500 Ω, and the rectification ratio is ~1 × 10 4 at a bias voltage of ±1 V (datasheet for BAT 62-02LS E6327 may be found on www.digikey.com ). High-frequency alternating current signals were generated by Keithley 3390 50 MHz arbitrary waveform generator. The input and output characterisation of the wireless coil were performed using an Agilent Infiniium DSO8104A oscilloscope (1 GHz, 4 channels). The wireless charging voltage and current to the battery were monitored using a BioLogic VMP3 electrochemical station. How to cite this article: Xu, S. et al . Stretchable batteries with self-similar serpentine interconnects and integrated wireless recharging systems. Nat. Commun. 4:1543 doi: 10.1038/ncomms2553 (2013).